Transcription errors induce proteotoxic stress and shorten cellular lifespan Transcription errors occur in all living cells; however, it is unknown how these errors affect cellular health. To answer this question, we monitor yeast cells that are genetically engineered to display error-prone transcription. We discover that these cells suffer from a profound loss in proteostasis, which sensitizes them to the expression of genes that are associated with protein-folding diseases in humans; thus, transcription errors represent a new molecular mechanism by which cells can acquire disease phenotypes. We further find that the error rate of transcription increases as cells age, suggesting that transcription errors affect proteostasis particularly in aging cells. Accordingly, transcription errors accelerate the aggregation of a peptide that is implicated in Alzheimer's disease, and shorten the lifespan of cells. These experiments reveal a previously unappreciated role for transcriptional fidelity in cellular health and aging. DNA replication, transcription and translation provide the foundation for life itself. Together, these three processes ensure the inheritance of our genome and the faithful expression of our genetic code. To preserve the integrity of this code, it is essential that these processes are carried out with remarkable precision. Sporadic errors are unavoidable though, and these errors reveal how important biological fidelity is for organismal health. For example, errors that occur during DNA replication contribute to carcinogenesis [1] , and errors that occur during translation contribute to amyloidosis [2] . How transcription errors affect cellular health is less well understood. Several experiments have now demonstrated though, that transcription errors have the potential to profoundly affect human health. For example, transcription errors in the gene that encodes the β-amyloid precursor protein generate toxic versions of the Aβ protein in patients with non-familial Alzheimer’s disease [3] , [4] . Similar transcription errors can generate toxic versions of the ubiquitin-B protein in patients with Down’s syndrome [3] , [4] , or activate oncogenic pathways in quiescent cells [5] . These transcription errors that occur at disease-related loci could directly contribute to human disease; however, underlying these specific, disease-related errors, is a much larger population of errors that occur randomly throughout the genome. How these random errors affect cellular health is completely unknown. Recently though, several alleles have been identified in the budding yeast Saccharomyces cerevisiae that result in error-prone transcription [6] , [7] . These alleles provide the first opportunity to fill this gap in our knowledge. Here, we monitored the health of two cell lines that exhibit error-prone transcription and demonstrate that random transcription errors profoundly affect cellular proteostasis, as well as the rate at which yeast cells age; thus, transcription errors represent a new molecular mechanism by which cells can acquire disease. 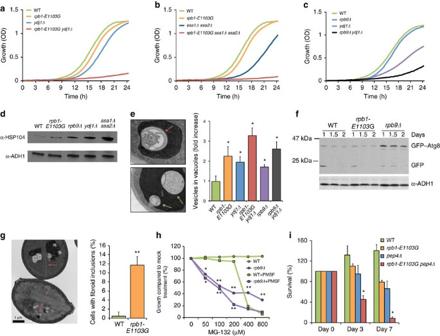Figure 1: Genetic, biochemical and ultrastructural evidence for proteotoxic stress. (a) In the absence ofYDJ1, rpb1-E1103G(MVY0001–4) cells grow very slowly. (b) In the absence ofYDJ1, rpb9Δcells grow very slowly (MVY0001, 3, 4 and 6). (c) In the absence ofSSA1andSSA2, rpb1-E1103Gcells grow very slowly (MVY0001, 2, 7 and 8). (d) Similar to cells that have lostYDJ1orSSA1andSSA2, rpb1-E1103Gcells andrpb9Δcells display increased expression of Hsp104 (MVY0001–4 and 7). (e) Autophagic remnants (top panel, red arrows) and inclusion bodies (middle panel, green arrows) are more frequently present in the vacuoles ofrpb1-E1103Gandrpb9Δcells compared with WT cells (MVY0001–6, micrograph taken from MVY0002). The prevalence of these vesicles can be exacerbated further byYDJ1deletion. Between 100 and 150 cells were examined for each genotype. (f)Rpb9Δcells display increased Atg8 expression. Cells were transformed with an N terminally GFP-tagged copy ofATG8and grown for the indicated number of days.Rpb9Δcells displayed a higher amount of Atg8 expression (top band) than WT cells and turn Atg8 over for a longer amount of time as they enter stationary phase (bottom band, indicating Atg8 cleaved from GFP in the vacuole; MVY0001–3). (g) Fibroid, crystalline protein aggregates (red arrows) are present inrpb1-E1103Gcells that were chronologically aged for 96 h in a 30 °C incubator (MVY0001–2). (h)Rpb9Δcells are more sensitive to increasing concentrations of MG-132 than WT cells. The sensitivity ofRpb9cells to MG-132 can be enhanced further by simultaneously inhibiting proteases present in the vacuole by 200 μM PMSF (MVY0001 and 3). Mock treatments included dimethylsulphoxide and ethanol, but not the drugs that were dissolved in them. (i) Deletion of PEP4 shortens the chronological lifespan ofrpb1-E1103Gcells (MVY0001, 2, 13 and 14). At least three biological replicates were used for each genotype for each experiment presented above. Images and western blots were quantified using the ImageJ software. All statistical analyses were performed with Prism software, using an unpaired, two-tailedt-test. All error bars indicate one s.d. from the mean. *P<0.05, **P<0.01. Upregulation of molecular chaperones in error-prone cells To determine how transcription errors affect cellular health, we monitored two cell lines that exhibit error-prone transcription (please see Supplementary Table 1 for a list of all the strains that are used in this manuscript). The first cell line carries a point mutation in the gene that encodes Rpb1 ( rpb1-E1103G , MVY0002), a core catalytic subunit of the RNA polymerase II complex [6] (RNAPII). The second cell line carries a deletion of the gene that encodes Rpb9 ( rpb9Δ, MVY0003), a non-essential subunit of the RNAPII complex [7] . These alleles display a 3–9-fold increase in the error rate of transcription in vivo and in vitro , and the mechanisms that are responsible for this increase are well established [6] , [7] , [8] , [9] , [10] . Interestingly, both of these cell lines exhibit a growth defect ( Fig. 1a,b ; Supplementary Fig. 1a ), suggesting that transcription errors have the potential to affect the overall health of a cell. To understand this observation, we used an unbiased mass spectrometry approach to identify proteins that were significantly upregulated in rpb1-E1103G and rpb9Δ cells compared with wild-type (WT) cells (MVY0001). In total, we detected 390 proteins. 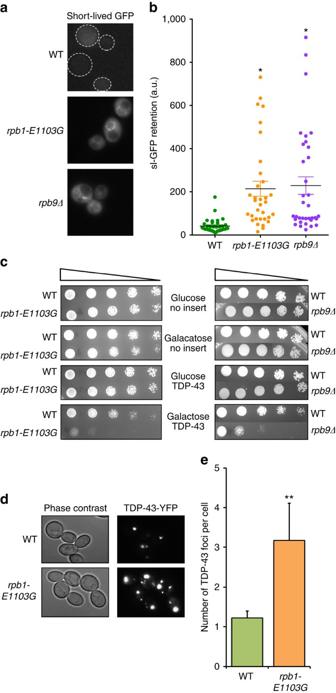Figure 2: Transcription errors overextend the protein quality control machinery. (a) Error-prone cells degrade a short-lived GFP (sl-GFP) molecule less efficiently than WT cells. WT cells andrpb1-E1103Gcells were transformed with a sl-GFP molecule, which is an indicator of the strain placed on cellular protein quality control pathways.rpb1-E1103Gandrpb9Δcells display a brighter GFP signal than WT cells, indicating that sl-GFP is degraded less efficiently in the error-prone cells compared with the WT cells and that PQC is overextended in the error-prone cells (MVY0001–3). (b) Quantification of the retention of sl-GFP in WT cells,rpb1-E1103Gcells andrpb9Δcells (MVY0001–3). (c) Error-prone cells are more sensitive to TDP-43 expression than WT cells. Cells were either transformed with an empty vector or a plasmid that contained a YFP-tagged copy of TDP-43, which was placed under the control of a GAL4 promoter. The transformed cells were then spotted in fourfold dilutions on the plates that contained gluocose (no expression) or galactose (expression). Expression of TDP-43 inhibited the growth ofrpb1-E1103Gandrpb9Δcells to a greater degree than WT cells, as shown by reduced growth of the error-prone cells at multiple dilutions (MVY0001–3). (d) Error-prone cells degrade TDP-43 less efficiently than WT cells. Cells were transformed with a YFP-tagged copy of TDP-43, grown into log-phase and monitored under a fluorescence microscope. Despite identical expression patterns,rpb1-E1103Gcells contain more protein aggregates than WT cells, indicating that they have greater difficulty destroying the TDP-43 protein. The aggregates inrpb1-E1103Gcells are also larger in size compared with WT cells (MVY0001–2). (e) Quantification of the number of TDP-43 foci in WT cells andrpb1-E1103Gcells. At least three biological replicates, and 100–150 cells were examined for each genotype for each experiment presented above. Images were quantified using the ImageJ software (MVY0001–2). All statistical analyses were performed with Prism software, using an unpaired, two-tailedt-test. Error bars inbindicate s.e. from the mean. Error bars ineindicate one s.d. from the mean. **P<0.01. Out of these 390 proteins, we found that 22 proteins were significantly upregulated ≥1.5-fold in the rpb1-E1103G cells, while 32 proteins were significantly upregulated ≥1.5-fold in the rpb9Δ cells ( Supplementary Table 2 ). Fifteen of these proteins were shared among the error-prone cell lines, and further analysis indicated that 7 of these play an important role in protein folding and protein quality control (PQC, Table 1A ). In addition, two chaperones were exclusively detected in the error-prone cells and not in the WT cells ( Table 1B ), which prohibited a quantitative comparison, while two additional chaperones were significantly upregulated in the rpb9Δ cells only ( Table 1C ). The upregulation of multiple chaperones in the error-prone cells suggests that they suffer from increased levels of proteotoxic stress. Figure 1: Genetic, biochemical and ultrastructural evidence for proteotoxic stress. ( a ) In the absence of YDJ1, rpb1-E1103G (MVY0001–4) cells grow very slowly. ( b ) In the absence of YDJ1, rpb9Δ cells grow very slowly (MVY0001, 3, 4 and 6). ( c ) In the absence of SSA1 and SSA2, rpb1-E1103G cells grow very slowly (MVY0001, 2, 7 and 8). ( d ) Similar to cells that have lost YDJ1 or SSA1 and SSA2, rpb1-E1103G cells and rpb9Δ cells display increased expression of Hsp104 (MVY0001–4 and 7). ( e ) Autophagic remnants (top panel, red arrows) and inclusion bodies (middle panel, green arrows) are more frequently present in the vacuoles of rpb1-E1103G and rpb9Δ cells compared with WT cells (MVY0001–6, micrograph taken from MVY0002). The prevalence of these vesicles can be exacerbated further by YDJ1 deletion. Between 100 and 150 cells were examined for each genotype. ( f ) Rpb9Δ cells display increased Atg8 expression. Cells were transformed with an N terminally GFP-tagged copy of ATG8 and grown for the indicated number of days. Rpb9Δ cells displayed a higher amount of Atg8 expression (top band) than WT cells and turn Atg8 over for a longer amount of time as they enter stationary phase (bottom band, indicating Atg8 cleaved from GFP in the vacuole; MVY0001–3). ( g ) Fibroid, crystalline protein aggregates (red arrows) are present in rpb1-E1103G cells that were chronologically aged for 96 h in a 30 °C incubator (MVY0001–2). ( h ) Rpb9Δ cells are more sensitive to increasing concentrations of MG-132 than WT cells. The sensitivity of Rpb9 cells to MG-132 can be enhanced further by simultaneously inhibiting proteases present in the vacuole by 200 μM PMSF (MVY0001 and 3). Mock treatments included dimethylsulphoxide and ethanol, but not the drugs that were dissolved in them. ( i ) Deletion of PEP4 shortens the chronological lifespan of rpb1-E1103G cells (MVY0001, 2, 13 and 14). At least three biological replicates were used for each genotype for each experiment presented above. Images and western blots were quantified using the ImageJ software. All statistical analyses were performed with Prism software, using an unpaired, two-tailed t -test. All error bars indicate one s.d. from the mean. * P <0.05, ** P <0.01. Full size image Table 1 Increased expression of molecular chaperones in error-prone cells. (A) List of all proteins that were significantly upregulated ≥1.5-fold in both rpb1-E1103G and rpb9Δ cells when compared with WT cells (MVY0001–3). (B) Molecular chaperones that were detected in the error-prone cells, but not in WT cells, so that a precise fold increase could not be calculated (MVY0001–3). (C) Molecular chaperones that were significantly upregulated in rpb9Δ cells, but not rpb1-E1103G cells. Full size table Molecular chaperones protect the health of error-prone cells To investigate this idea further, we used genetics, biochemistry, fluorescence microscopy and electron microscopy to find additional evidence for proteotoxic stress in the error-prone cells. First, we used a genetic approach to test whether molecular chaperones are indeed critical for the health of the error-prone cells. To this end, we introduced a YDJ1 deletion into the error-prone cells using a standard mating and sporulation approach. YDJ1 encodes an Hsp40 co-chaperone that contributes to the folding process of nascent proteins, and helps refold proteins that were previously misfolded [11] . In the absence of YDJ1 , we found that rpb1-E1103G (MVY0005) and rpb9Δ cells (MVY0006) produce exceptionally small colonies ( Supplementary Fig. 1a ), grow at a slow rate ( Supplementary Fig. 1a, b ), and exhibit a swollen appearance ( Supplementary Fig. 1b ). Taken together, these results indicate that YDJ1 is critical for the overall health of cells that display error-prone transcription. To determine whether this finding was unique to YDJ1 , or whether it could be extended to other chaperones, we also deleted SSA1 and SSA2 in rpb1-E1103G cells. Ssa1 and Ssa2 are two chaperones that are in the Hsp70 family [11] and are 98% identical. Accordingly, they need to be deleted simultaneously in WT cells to affect cellular function (MVY0007). We found that the growth rate of rpb1-E1103G ssa1Δ ssa2Δ cells (MVY0008) closely resembles the growth rate of rpb1-E1103G ydj1Δ cells ( Fig. 1c ), and that the rpb1-E1103G ssa1Δ ssa2Δ cells exhibit a similar swollen appearance. Rpb9Δ cells, and to a lesser degree rpb1-E1103G cells, were also more sensitive to inhibition of Hsp82 with radicicol [12] than WT cells ( Supplementary Fig. 2 ). Hsp82 is a key molecular chaperone that is upregulated in response to heat and stress [13] and contributes to the folding process of a specific set of proteins that is particularly difficult to fold [14] . Thus, multiple chaperones in addition to Ydj1 are required to maintain the health of the error-prone cells, supporting the hypothesis that these cells suffer from proteotoxic stress. The error-prone cells suffer from proteotoxic stress To find additional evidence for the presence of proteotoxic stress in the error-prone cells, we monitored the expression of Hsp104 ( Fig. 1d ), a protein that disassembles protein aggregates, and whose upregulation is a common response to proteotoxic stress and protein aggregation [15] . We found that rpb1-E1103G and rpb9Δ cells indeed exhibit increased expression of Hsp104 compared with WT cells, similar to cells that are known to experience proteotoxic stress due to loss of YDJ1 (MVY0004) or SSA1 and SSA2 (ref. 15 ; MVY0007, Fig. 1d ). This observation was confirmed in vivo using fluorescent imaging of a green fluorescent protein (GFP)-tagged copy of HSP104 , which was chromosomally integrated into WT (MVY0009), rpb1-E1103G (MVY0010) and rpb9Δ cells (MVY0011, Supplementary Fig. 3 ). The upregulation of Hsp104 indicates that despite the efforts of multiple molecular chaperones, protein aggregation may be occurring to a greater degree in the error-prone cell lines. Protein aggregates and other forms of proteotoxic stress are frequently cleared from cells by autophagy and vacuolar degradation. Accordingly, we found that rpb1-E1103G cells and rpb9Δ cells contain more autophagic vesicles inside their vacuoles than WT cells ( Fig. 1e ), indicating increased autophagic activity ( Fig. 1e ). Although it is difficult to distinguish between microautophagy, macroautophagy and cytoplasm-to-vacuole targeting from these images, we found that quarter of these vesicles contained condensed multilammelar remnants that are indicative of macroautophagy ( Supplementary Fig. 4a ). Accordingly, we observed more multilammelar inclusions inside the vacuoles of the error-prone cells when YDJ1 was deleted (MVY0005, Fig. 1e ) and less when ATG1 was deleted (MVY0012), a gene that is important for phagophore formation ( Supplementary Fig. 4a ). In addition, rpb9Δ cells display increased expression of Atg8, a key component of the macroautophagy and the cytoplasm-to-vacuole targeting pathway ( Fig. 1f ). Autophagy is especially important for the long-term health of the error-prone cells, as deletion of ATG6 or VAC8 reduced the lifespan of rpb1-E1103G cells ( Supplementary Fig. 4b–c ). Finally, we found direct evidence for protein aggregation in chronologically aged rpb1-E1103G cells, which accumulated fibroid, crystalline protein aggregates inside their cytoplasm that could span the length of an entire cell ( Fig. 1g ). Cells can degrade autophagic debris and toxic proteins with proteases that are located in the proteasome and the vacuole. To test the importance of these proteases for the health of the error-prone cells, we treated WT cells and error-prone cells with MG-132, a drug that inhibits the proteasome [16] , and PMSF, a drug that inhibits proteases present in the vacuole [17] . We found that rpb9Δ cells exhibit a greatly increased sensitivity to MG-132 ( Fig. 1h ) and PMSF compared with WT cells, and a combination of these two drugs was the most effective ( Fig. 1g ). Although these drugs did not significantly reduce the growth rate of the rpb1-E1103G cells, we found that deletion of PEP4 (which encodes a key protease inside the vacuole [18] ) in the rpb1-E1103G cells, greatly diminished the lifespan of rpb1-E1103G cells (MVY0014, Fig. 1i ), indicating that protease activity is also important for the health of rpb1-E1103G cells, although it is not important enough to affect the rate at which the cells grow. The combined weight of all of these experiments strongly suggests that the error-prone cells suffer from increased levels of proteotoxic stress compared with WT cells. The enhanced growth defect of rpb9Δ cells, in combination with their enhanced sensitivity to PMSF, MG-132 and Hsp82 inhibition, as well as their enhanced induction of Hsp104 and Atg8, further suggest that rpb9Δ cells suffer from greater amounts of proteotoxic stress than rpb1-E1103G cells. Interestingly, rpb9Δ cells are also highly sensitive to deletion of UPF1 , 2 or 3 (MV0015-MV0017, Supplementary Fig. 5 ), three genes that play an essential role in the nonsense-mediated RNA decay (NMD) pathway. NMD provides a way for cells to control the quality of the transcriptome, by degrading messenger RNA (mRNA) molecules that contain a premature stop codon [19] . Since frameshifts are the most common source of premature stop codons, this observation suggests that rpb9Δ cells commit a greater number of frameshift errors than rpb1-E1103G cells, which could help explain why they suffer from an increased level of proteotoxic stress. It is important to note though, that in contrast to the rpb1-E1103G allele, deletion of RPB9 also results in a measurable effect on transcription itself [7] . This perturbation could contribute to the increased level of proteotoxic stress in rpb9Δ cells as well. Transcription errors potentiate toxic misfolded proteins Recent evidence indicates that the capacity of cells to combat proteotoxic stress is limited. For example, the expression of an aggregation-prone version of the Huntingtin protein (a human protein that causes a neuromuscular disorder [20] ) in Caenorhabditis elegans overwhelms the capacity of the PQC machinery to such an extent that regular maintenance tasks (such as assisting with the folding process of endogenous proteins) are neglected [21] . 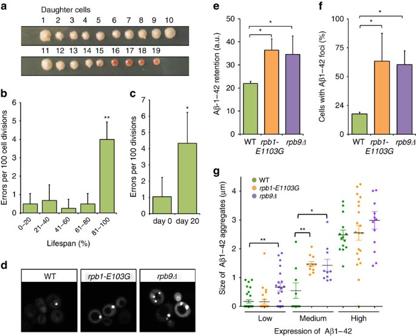Figure 3: The fidelity of transcription changes as a function of age. (a) Example of a replicative assay for one mother cell. Daughter cells were collected from an aging mother cell, displayed in a row across a plate and allowed to grow into colonies. If a transcription error occurred in the mother cell, all subsequent daughter cells born after this event would grow into red colonies (daughter 16–19). If a transcription error occurred in the daughter cell though, then only that colony would be affected (daughter 15) (diploid cross between GRY3337 and GRY3724). (b) The error rate of transcription increases approximately eightfold as a function of the replicative age of the cell. (c) The error rate of transcription increases approximately fourfold as a function of the chronological age of the cell. (d) Aβ1-42 aggregates into more numerous foci inrpb1-E1103Gandrpb9Δcells than in WT cells. Dashed outlines indicate cells that are difficult to see due to low fluorescence (MVY0001–3). (e) More Aβ1-42 is present insiderpb1-E1103Gcompared with WT cells despite equal expression levels; however,rpb9Δcells have a 20% lower expression of Aβ1-42 compared with WT cells. We therefore normalized Aβ1-42 expression inrpb9Δcells to GFP expression. With or without this correction, more Aβ1-42 is retained inside both of the error-prone cells compared with WT cells. Approximately 120 cells were analysed for each genotype (MVY0001–3). (f) A greater number of Aβ1-42 foci appear inrpb1-E1103Gandrpb9Δcells (MVY0001–3). (g) Aβ1-42 starts to aggregate at lower levels of expression inrpb1-E1103Gandrpb9Δcells compared. This threshold is reached first inrpb9Δcells, and then in therpb1-E1103Gcells. At least three biological replicates were used for each genotype for each experiment presented above. Images were quantified using the ImageJ software (MVY0001–3). All statistical analyses were performed with Prism software, using an unpaired, two-tailedt-test. Error bars inFig. 2b,c,e,findicate one s.d. from the mean. Error bars inFig. 2gindicate s.e. from the mean. *P<0.05, **P<0.01. To test whether error-prone transcription could overwhelm the PQC machinery in a similar manner, we monitored the status of the PQC machinery with a plasmid that contains a fluorescent reporter protein (for a list of all plasmids used in this manuscript, please see Supplementary Table 3 ). This reporter protein consists of a short-lived GFP molecule (sl-GFP) that is a target for destruction by the proteasome [22] . Retention of sl-GFP inside a cell is therefore a barometer for the workload of the PQC machinery [22] . Notably, rpb1-E1103G and rpb9Δ cells retain more sl-GFP than WT cells ( Fig. 2a,b ), which reinforces the idea that rpb1-E1103G cells suffer from proteotoxic stress and indicates that the PQC machinery is indeed overextended. To explore this idea further, we expressed a YFP-tagged copy of TDP-43 in the error-prone cells [23] , a toxic protein that causes amyotrophic lateral sclerosis. Although TDP-43 is only slightly toxic in WT cells, we noticed that the viability of rpb1-E1103G and rpb9Δ cells was greatly diminished by TDP-43 ( Fig. 2c ). We observed a similar phenomenon when we overexpressed a toxic repeat of 17 alanines in the rpb1-E1103G cells, while a non-toxic control containing a repeat of 8 alanines did not affect cellular viability ( Supplementary Fig. 6a ). The increased toxicity of TDP-43 was also apparent at the molecular level, as a fluorescently tagged copy of TDP-43 aggregated into larger and more numerous foci in rpb1-E1103G cells compared with WT cells ( Fig. 2d,e ). These results indicate that WT cells degrade TDP-43 more efficiently than error-prone cells, mirroring our results with sl-GFP ( Fig. 2a ). Figure 2: Transcription errors overextend the protein quality control machinery. ( a ) Error-prone cells degrade a short-lived GFP (sl-GFP) molecule less efficiently than WT cells. WT cells and rpb1-E1103G cells were transformed with a sl-GFP molecule, which is an indicator of the strain placed on cellular protein quality control pathways. rpb1-E1103G and rpb9Δ cells display a brighter GFP signal than WT cells, indicating that sl-GFP is degraded less efficiently in the error-prone cells compared with the WT cells and that PQC is overextended in the error-prone cells (MVY0001–3). ( b ) Quantification of the retention of sl-GFP in WT cells, rpb1-E1103G cells and rpb9Δ cells (MVY0001–3). ( c ) Error-prone cells are more sensitive to TDP-43 expression than WT cells. Cells were either transformed with an empty vector or a plasmid that contained a YFP-tagged copy of TDP-43, which was placed under the control of a GAL4 promoter. The transformed cells were then spotted in fourfold dilutions on the plates that contained gluocose (no expression) or galactose (expression). Expression of TDP-43 inhibited the growth of rpb1-E1103G and rpb9Δ cells to a greater degree than WT cells, as shown by reduced growth of the error-prone cells at multiple dilutions (MVY0001–3). ( d ) Error-prone cells degrade TDP-43 less efficiently than WT cells. Cells were transformed with a YFP-tagged copy of TDP-43, grown into log-phase and monitored under a fluorescence microscope. Despite identical expression patterns, rpb1-E1103G cells contain more protein aggregates than WT cells, indicating that they have greater difficulty destroying the TDP-43 protein. The aggregates in rpb1-E1103G cells are also larger in size compared with WT cells (MVY0001–2). ( e ) Quantification of the number of TDP-43 foci in WT cells and rpb1-E1103G cells. At least three biological replicates, and 100–150 cells were examined for each genotype for each experiment presented above. Images were quantified using the ImageJ software (MVY0001–2). All statistical analyses were performed with Prism software, using an unpaired, two-tailed t -test. Error bars in b indicate s.e. from the mean. Error bars in e indicate one s.d. from the mean. ** P <0.01. Full size image To determine the breadth of these observations, we expressed two additional proteins in the error-prone cells: the toxic glutamine repeat region of the Huntingtin protein, and the yeast prion Rnq1 (ref. 24 ). These proteins form amyloid-like aggregates that are structurally distinct from the amorphous aggregates of TDP-43 and alanine repeats [25] . Despite this mechanistic difference though, we found that Rnq1 and a toxic version of the Huntingtin protein (Htt103Q) greatly reduced the viability of rpb9Δ cells compared with WT cells, whereas a benign version of Huntingtin (Htt25Q) did not ( Supplementary Fig. 6b ). However, Htt103Q and Rnq1 did not affect rpb1-E1103G cells more than WT cells, which demonstrate that rpb9Δ cells have a wider sensitivity to toxic proteins than rpb1-E1103G cells, consistent with the observation that rpb9Δ cells suffer from a greater amount of proteotoxic stress. Taken together, these results indicate that transcription errors can overextend the PQC machinery, which allows toxic proteins that are associated with disease to escape degradation, thereby enhancing their toxicity and rate of aggregation. Transcription errors increase with age Proteotoxic stress is a universal hallmark of aging cells [26] . However, the molecular mechanisms that cause proteotoxic stress in aging cells remain unknown. Since transcription errors induce proteotoxic stress, we wondered whether transcription errors could represent one of these mechanisms. To test this possibility, we measured the transcriptional error rate of WT cells as a function of age. For these measurements, we used an assay that records transcription errors on a track of 10 cytosines [6] as red sectors in growing colonies ( Fig. 3a ). This cytosine track places the gene that encodes Cre-recombinase out of frame. If RNAPII slips on this track and reinstates the proper reading frame, active proteins are generated. Cre-recombinase then excises a target elsewhere in the genome, which results in the accumulation of red pigment inside the cells. As a result, a temporary transcription error is converted into a tractable, genetic mutation. To determine whether aging affects the transcriptional error rate, we aged these reporter cells (a cross between GRY3337 and GRY3724) replicatively and chronologically: the replicative lifespan of yeast cells is measured by the number of daughter cells that are born from a single mother cell, and is thought to be a model for the lifespan of mitotic cells, whereas the chronological lifespan is measured by the time a cell can stay alive in a non-dividing state, which is thought to be a model for the lifespan of post-mitotic cells [27] . We discovered that the error rate of transcription increases ≈8-fold in the final stages of the replicative lifespan of the cells ( Fig. 3b ), and 4–10-fold during their chronological lifespan ( Fig. 3c ; Supplementary Fig. 7 ). We confirmed that these events were the result of transcription errors and not genetic mutations in two ways. First, we sequenced the Cre-locus to search for genetic mutations, but found none in the 48 clones we tested. Second, we sporulated cells that were derived from the red colonies and mated them to a second reporter. If a genetic error had reactivated Cre-recombinase, these cells would continuously express an active version of Cre-recombinase and activate the second reporter immediately. However, no Cre-activity was detected in any of the 48 clones tested. As a result of the increased number of transcription errors in aging cells, we conclude that transcription errors place an increasing burden on the PQC of the aging cells, which suggests that transcription errors are partially responsible for the increased levels of proteotoxic stress seen in aging cells. In humans, this decline in proteostasis predisposes cells to age-related pathology that is mediated by toxic proteins, as seen in Alzheimer’s and Parkinson’s disease [26] . To specifically test whether transcription errors are capable of modulating the degradation of proteins that are associated with age-related diseases, we expressed a GFP-tagged copy of Aβ1-42 in our cell lines. Aβ1-42 is an aggregation-prone, short peptide, which forms large amyloid plaques in Alzheimer’s patients, and is a powerful target for cellular PQC. Similar to TDP-43, we found that Aβ1-42 is destroyed less efficiently in rpb1-E1103G and rpb9Δ cells compared with WT cells ( Fig. 3d,e ), and aggregates into larger, more numerous foci in the error-prone cells ( Fig. 3f ). The aggregation of Aβ1-42 strongly depends on the level of expression, and we found that aggregation of Aβ1-42 is initiated at lower levels of expression in the error-prone cells compared with the WT cells ( Fig. 3g ). Taken together, these experiments indicate that transcription errors increase with age in yeast, and that these errors can affect the degradation and aggregation of proteins that are associated with age-related diseases in humans. Figure 3: The fidelity of transcription changes as a function of age. ( a ) Example of a replicative assay for one mother cell. Daughter cells were collected from an aging mother cell, displayed in a row across a plate and allowed to grow into colonies. If a transcription error occurred in the mother cell, all subsequent daughter cells born after this event would grow into red colonies (daughter 16–19). If a transcription error occurred in the daughter cell though, then only that colony would be affected (daughter 15) (diploid cross between GRY3337 and GRY3724). ( b ) The error rate of transcription increases approximately eightfold as a function of the replicative age of the cell. ( c ) The error rate of transcription increases approximately fourfold as a function of the chronological age of the cell. ( d ) Aβ1-42 aggregates into more numerous foci in rpb1-E1103G and rpb9Δ cells than in WT cells. Dashed outlines indicate cells that are difficult to see due to low fluorescence (MVY0001–3). ( e ) More Aβ1-42 is present inside rpb1-E1103G compared with WT cells despite equal expression levels; however, rpb9Δ cells have a 20% lower expression of Aβ1-42 compared with WT cells. We therefore normalized Aβ1-42 expression in rpb9Δ cells to GFP expression. With or without this correction, more Aβ1-42 is retained inside both of the error-prone cells compared with WT cells. Approximately 120 cells were analysed for each genotype (MVY0001–3). ( f ) A greater number of Aβ1-42 foci appear in rpb1-E1103G and rpb9Δ cells (MVY0001–3). ( g ) Aβ1-42 starts to aggregate at lower levels of expression in rpb1-E1103G and rpb9Δ cells compared. This threshold is reached first in rpb9Δ cells, and then in the rpb1-E1103G cells. At least three biological replicates were used for each genotype for each experiment presented above. Images were quantified using the ImageJ software (MVY0001–3). All statistical analyses were performed with Prism software, using an unpaired, two-tailed t -test. Error bars in Fig. 2b,c,e,f indicate one s.d. from the mean. Error bars in Fig. 2g indicate s.e. from the mean. * P <0.05, ** P <0.01. Full size image Transcription errors decrease the lifespan of cells In addition to age-related pathology, proteotoxicity also contributes to the mortality of aging cells [28] ; thus, transcription errors may affect the lifespan of cells as well. To investigate this possibility, we monitored the replicative and chronological lifespan of rpb1-E1103G and rpb9Δ cells, and found that these cell lines exhibit a shorter replicative and chronological lifespan compared with WT cells ( Fig. 4a,b ). The lifespan of the error-prone cells could be shortened further by exacerbating the level of proteotoxic stress through YDJ1 or SSA1 and SSA2 deletion ( Fig. 4c,d ; Supplementary Fig. 8 ), or by compromising RNA quality control (RQC) through UPF1 deletion ( Supplementary Fig. 8 ). After determining how transcription errors affect aging cells, we decided to investigate whether these effects are permanent, or reversible. Because dietary restriction delays the onset of age-related pathology and extends the replicative lifespan of cells [29] , we tested whether dietary restriction could also reverse the deleterious effects of transcription errors on the lifespan of aging cells. To do this, we monitored the replicative lifespan of error-prone cells that were grown on normal (2%) or restricted concentrations of glucose. Importantly, restricting glucose to 0.05, 0.1 or 0.15% rescued the lifespan of both rpb1-E1103G and rpb9Δ cells ( Fig. 4e,f ; Supplementary Fig. 9a, b ), which demonstrates that the deleterious effects of transcription errors on the lifespan of aging cells can indeed be reversed. Furthermore, the lifespan extension of the error-prone cells depended on the presence of YDJ1 and SSA1 and SSA2 ( Fig. 4e,f , Supplementary Fig. 9c–d ), indicating that this extension is orchestrated by the manipulation of PQC pathways, a well-known effect of dietary restriction [30] . To determine whether the chronological lifespan of the error-prone cells could be rescued as well, we treated the error-prone cells with rapamycin, a drug that extends the chronological lifespan of WT yeast cells by modulating autophagy and protein translation [31] . Rapamycin also extends the lifespan of mice and contributes to the health of aging mice [31] , [32] , [33] . Interestingly, rapamycin could extend the chronological lifespan of the error-prone cells as well, and partially rescued the replicative lifespan of the rpb1-E1103G cells ( Fig. 4g,h ). 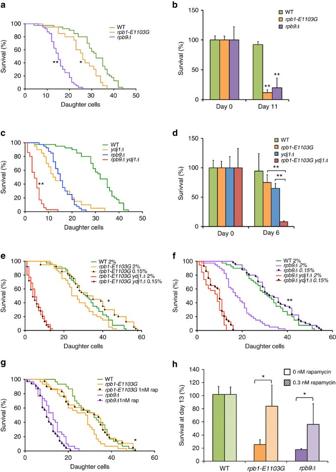Figure 4: Error-prone cells have a shortened lifespan. (a)rpb1-E1103Gandrpb9Δcells live shorter replicative lifespans than WT cells. For example, the average lifespan of WT cells is ≈30 divisions, while the average lifespan ofrpb9Δcells is ≈18 divisions. In all replicative lifespan assays, the lifespan of 20–40 mother cells was measured per sample (MVY0001–3). (b)rpb1-E1103Gandrpb9Δcells live shorter chronological lifespans than WT cells. For all chronological lifespan assays, the lifespan of 3–5 replicates was measured per sample (MVY0001–3). (c) Deletion ofYDJ1results in a profound reduction of the replicative lifespan ofrpb1-E1103Gcells (MVY0001, 2, 4 and 5). (d) Deletion ofYDJ1results in a profound reduction of the chronological lifespan ofrpb1-E1103Gcells (MVY0001, 2, 4 and 5). (e) Dietary restriction rescues the shortened lifespan ofrpb1-E1103Gcells, but notrpb1-E1103G ydj1Δcells (MVY0001, 2 and 5). (f) Dietary restriction rescues the shortened lifespan of rpb9Δ cells, but notrpb9Δ ydj1Δcells (MVY0001, 3 and 6). (g) Rapamycin partially rescues the replicative lifespan ofrpb1-E1103Gcells, but notrpb9Δcells. (h) Rapamycin rescues the chronological lifespan ofrp1-E1103Gcells andrpb9Δcells. At least three biological replicates were used for each genotype for each experiment presented above. Kaplan–Meier curves and analysis were performed using the Prism Graphpad software. All statistical analyses on the chronological lifespan of cells were performed with Prism software, using an unpaired, two-tailedt-test. Error bars indicate one s.d. from the mean. All statistical analyses on the replicative lifespan of cells were performed with Prism software, using a curve comparison, log rank (Mantel–Cox) test. *P<0.05, **P<0.01. Figure 4: Error-prone cells have a shortened lifespan. ( a ) rpb1-E1103G and rpb9Δ cells live shorter replicative lifespans than WT cells. For example, the average lifespan of WT cells is ≈30 divisions, while the average lifespan of rpb9Δ cells is ≈18 divisions. In all replicative lifespan assays, the lifespan of 20–40 mother cells was measured per sample (MVY0001–3). ( b ) rpb1-E1103G and rpb9Δ cells live shorter chronological lifespans than WT cells. For all chronological lifespan assays, the lifespan of 3–5 replicates was measured per sample (MVY0001–3). ( c ) Deletion of YDJ1 results in a profound reduction of the replicative lifespan of rpb1-E1103G cells (MVY0001, 2, 4 and 5). ( d ) Deletion of YDJ1 results in a profound reduction of the chronological lifespan of rpb1-E1103G cells (MVY0001, 2, 4 and 5). ( e ) Dietary restriction rescues the shortened lifespan of rpb1-E1103G cells, but not rpb1-E1103G ydj1Δ cells (MVY0001, 2 and 5). ( f ) Dietary restriction rescues the shortened lifespan of rpb9Δ cells, but not rpb9Δ ydj1Δ cells (MVY0001, 3 and 6). ( g ) Rapamycin partially rescues the replicative lifespan of rpb1-E1103G cells, but not rpb9Δ cells. ( h ) Rapamycin rescues the chronological lifespan of rp1-E1103G cells and rpb9Δ cells. At least three biological replicates were used for each genotype for each experiment presented above. Kaplan–Meier curves and analysis were performed using the Prism Graphpad software. All statistical analyses on the chronological lifespan of cells were performed with Prism software, using an unpaired, two-tailed t -test. Error bars indicate one s.d. from the mean. All statistical analyses on the replicative lifespan of cells were performed with Prism software, using a curve comparison, log rank (Mantel–Cox) test. * P <0.05, ** P <0.01. Full size image Basic biological consequences of transcription errors The genome provides a precise, biological blueprint of life. To implement this blueprint correctly, the genome must be read with great precision; however, due to the constraints of biological fidelity, it is impossible for this process to be completely error free. As a result, transcription errors can occur at any time, in any transcript, and how these random errors affect cellular health is unknown. Here we answer this question by studying cells that express an error-prone version of RNAPII, and we demonstrate that transcription errors affect cellular health by inducing proteotoxic stress. Most likely, this increase in proteotoxic stress is caused by transcription errors that change structurally important amino acids in polypeptide chains. For example, a transcription error that replaces a hydrophobic amino acid with a hydrophilic amino acid could substantially distort the folding process of a protein. Similar distortions are caused by genetic mutations [34] and translation errors [2] . These experiments expose a surprising new role for PQC in living cells: to counteract the deleterious effects of transcription errors. Eukaryotic cells also contain two major RQC pathways: NMD and nonstop mRNA decay. NMD degrades mRNA molecules that contain a premature stop codon, while nonstop mRNA decay degrades molecules that lack a stop codon altogether [19] . The need for PQC to complement these pathways indicates that RQC alone is not sufficient to protect cells from transcription errors. One limitation is that most single-base substitutions do not generate a premature stop codon, or affect an existing stop codon. As a result, these errors are virtually undetectable by RNA quality control. Alternatively, transcription errors could also evade the RQC machinery by overwhelming its capacity, which is an important possibility for frameshift errors. We suspect that both of these mechanisms contribute to the proteotoxic stress that is experienced by the error-prone cells. We further found that transcription errors have the potential to affect cells in a medically relevant manner by encumbering the PQC machinery, which allows disease-related proteins to escape degradation, thereby increasing their toxicity; thus, randomly occurring transcription errors represent a new molecular mechanism by which cells can acquire disease. We also discovered that the error rate of transcription increases with age in yeast, which contributes to the decline in proteostasis seen in aging cells. As a result, transcription errors allow toxic proteins to escape the PQC machinery particularly in aging cells. In humans, an age-related increase in the error rate of transcription could allow proteins associated with age-related diseases such as Alzheimer’s and Parkinson’s disease to accumulate in aging neurons and increase cellular mortality, which would provide valuable new insight into the molecular aetiology of numerous age-related diseases and the mechanisms by which dietary restriction and rapamycin promote healthy aging. To test this possibility, it will be important to produce animal models and human cell lines that display error-prone transcription. The potential link between neurons and transcription errors is especially intriguing because oxidative damage is a powerful source of transcription errors. As oxidative damage accumulates in aging neurons, it could raise the transcriptional error rate and facilitate the onset of age-related diseases. Accordingly, transcription errors may represent a molecular link between aging and age-related diseases. In theory though, any form of DNA damage could contribute to the transcriptional error rate, including most of the mutagens we are currently aware of. If so, we may be substantially underestimating the harmful effects mutagens have on cellular health. By taking advantage of recently developed next-generation sequencing technology, it may be possible to test this hypothesis. Alternatively, mutagens could also damage ribonucleotides directly, which could alter the fidelity with which they are incorporated during transcription, or lower the fidelity of translation. DNA-damaging reagents are especially dangerous though, because they can cause repeated transcription errors at a single base [5] , [35] , [36] . These errors can generate a large number of proteins with a single, potentially harmful mutation. For example, transcription errors that occur repeatedly in the gene that encodes the amyloid precursor protein generate toxic versions of the Aβ protein in Alzheimer’s patients [3] , [4] . A remarkable prediction from our observations is therefore that an age-related increase in transcription errors may not only result in highly specific, disease-related proteins, but also provide the very conditions that allow these proteins to escape the surveillance of the PQC machinery. Cell strains and plasmids All the strains that were used for our experiments were backcrossed 15 times into the BY4742/BY4741 background, directly pulled from the BY4742 MATα knockout collection, or sporulated from the BY4743 heterozygous knockout collection to create haploid cells in the BY4742/BY4741 background. Unless otherwise noted, WT cells, rpb1-E1103 cells or rpb9Δ cells refer to MVY0001, MVY0002 or MVY0003, respectively. All other strains are specifically referred to with genotype and strain number in the text. In addition, each figure legend contains information about the exact strains that were used to acquire the data that is depicted. Double mutants were generated using standard mating and sporulation protocols using the BY4742 MATα knockout collection from Open Biosystems as a source for the deletions of key genes. For instance, to delete a single gene in a WT or error-prone background, we crossed rpb1-E1103G or rpb9Δ cell lines into the appropriate strain from the MATα knockout collection. The diploid cells were then sporulated, microdissected and genotyped so that each strain was known to posses the desired auxotrophy markers (see strain list). All the plasmids used for our experiments were previously generated, and no modifications were made. All plasmid transformations were performed using standard lithium acetate protocols. Lifespan experiments Replicative lifespan assays were performed as previously reported. Briefly, single colonies were streaked out on fresh YAPD plates, grown overnight and restreaked onto a new YAPD plate in the morning. After 6 h of growth, a small amount of cells was moved onto a fresh, experimental plate, and 20–60 mother cells were displayed for each genotype. The daughters, or the grand daughters of these cells, were used for our lifespan assays, so that each cell was a virgin at the start of the experiment. Chronological aging assays were performed by inoculating single colonies grown on YAPD plates into 3 ml of YAPD medium. These cultures were grown overnight, and diluted 10-fold into fresh YAPD medium the next morning. This culture was then allowed to grow uninterrupted for 48 h to drive the cells into stationary phase. After 48 h, the number of colony-forming units (CFUs) present in the culture was determined by diluting the cells in water, and plating them on freshly made YAPD plates. Three, 7, 10 and 14 days later, the number of CFUs was assessed again and compared with the 48-h time point to calculate survival. The survival of each genotype was monitored in triplicate or quadruplicate, starting from a unique, single colony. Western blotting Single colonies were inoculated in YAPD, grown overnight and then diluted in fresh YAPD the next morning. The cells were then cultured until they reached log-phase, and 2 ODs from each cell line were collected and suspended in 100 μl of SDS loading buffer adapted for cellular lysis, supplemented with 100 μl of acid washed glass beads. The cells were then boiled immediately for 30 s, and subsequently vortexed for 30 s to lyse them. These boiling and vortexing steps were repeated four more times to fully lyse the cells. Then, 50 μl of loading buffer was added to the lysates, which was spun down to pellet large cell debris. After centrifugation, the protein lysate was immediately loaded onto a 4–12% gel and blotted for the appropriate antibody after transfer onto a nitrocellulose membrane. The membrane was scanned using Typhoon imager system. The rabbit polyclonal HSP104 antibody was purchased from Abcam (ab69549, 1:5,000), rabbit polyclonal adh1 antibody was bought from Abcam (ab80354, 1:2,000) and the goat anti rabbit secondary antibody, conjugated with Alexafluor 488, was purchased from Invitrogen and Molecular Probes. For monitoring autophagy by GFP–ATG8 induction, GFP–ATG8 was expressed from its endogenous promoter using pRS316GFP-aut7 (ref. 37 ; Atg8). Cells were inoculated from three independent log-phase starter cultures at 0.008 OD 600 and incubated at 30 °C in an orbital shaker. At indicated time points, 2.0 OD 600 were collected and subjected to immunoblot analysis as described previously [38] . GFP–ATG8 induction was determined from the ratio of the signal intensity of full-length GFP–ATG8 to the signal intensity of the lysis control ADH1. The monoclonal anti-GFP antibody was purchased from Santa Cruz (B-2, 1:5,000). Resulting ratios were normalized to WT day 1 signal to adjust for signal intensity variation between different immunoblot membranes. A two-tailed Student’s t -test was applied to the resulting values to determine the statistical significance. Electron microscopy Yeast cells were prepared for transmission electron microscopy using a modification of methods published previously [39] . Specifically, cells were fixed with 2% glutaraldehyde in 0.1 M PIPES buffer, pH 6.8, containing 1 mM MgCl 2 , 1 mM CaCl 2 and 0.1 M sorbitol for overnight at 4 ˚C. Following cell wall permeabilization with 1% sodium metaperiodate, the cell pellets were post-fixed for 1 h with 1% osmium tetroxide/1.25% potassium ferrocyanide/0.1 M PIPES buffer, pH 6.8, and stained en bloc in 2% aqueous uranyl acetate for 20 min. The pellets were dehydrated using an increasing ethanol series followed by propylene oxide and embedment in Spurr’s epoxy resin (Electron Microscopy Sciences, Hatfield, PA). Ultrathin sections (70 nm) were cut and mounted on 200 mesh copper grids and stained with Reynolds’ lead citrate [40] . The sections were observed at 80 kV using a LEO EM910 transmission electron microscope (Carl Zeiss Microscopy, LLC, Thornwood, NY) and digital images were taken using a Gatan Orius SC1000 digital camera with Digital Micrograph 3.11.0 software (Gatan, Inc., Pleasanton, CA). Protein digestion for mass spectrometry WT, rpb1-E1103G and rpb9Δ cells were pulverized and frozen (−80 °C) until further use. Each sample contained three biological replicates. Lysed lyophilized cells were suspended in 50 mM ammonium bicarbonate with protease inhibitors (Roche cOmplete Protease Inhibitor Cocktail) prepared to manufacturer’s recommendations. Protein concentrations were determined via a Coomassie Plus (Bradford) Assay Kit (Thermo Scientific, 23236) with bovine serum albumin standard. Samples for digestion were diluted with 50 mM ammonium bicarbonate to provide equivalent protein concentration in all samples. A standard in-solution tryptic digestion protocol ( http://www.genome.duke.edu/cores/proteomics/sample-preparation/ ) was followed for shotgun digestion of all samples. In short, Rapigest SF acid-labile surfactant (Waters Corporation, Milford, MA) was added to 50 μg of protein to a final concentration of 0.1%. Samples were vortexed, heated at 40 °C for 10 min and centrifuged to condensate. Dithiothreitol (Sigma-Aldrich Co., St. Louis, MO) was added to a final concentration of 10 mM to reduce disulfide bonds. Samples were vortexed and heated to 80 °C for 15 min. All samples were then cooled, centrifuged to condensate and iodoacetamide (Sigma-Aldrich Co.) was added to a final concentration of 20 mM to alkylate disulfide bonds. The samples were incubated in the dark for 30 min before trypsin (TPCK-modified, Sigma-Aldrich Co.) was added in a 1:50 trypsin to protein ratio. Digestion occurred overnight at 37 °C, followed by acidification with trifluoroacetic acid (Sigma-Aldrich Co.) to 1.0% by volume. Samples were then centrifuged (22,000 g ) for 5 min and the supernatant was transferred into total recovery vials. For quantification, bovine serum albumin digest (Waters Corporation, 186002329) was added as an internal standard at a concentration of 25 fmol μl −1 . Liquid chromatography and mass spectrometry analysis Each sample was injected (2 μl) onto a RPLC-MS/MS Waters nanoAcquity/SynaptG2 system. Samples were initially trapped on a 5 mm × 180 μm trap column packed with 5 μm Symmetry C18 particles (Waters) at a flow rate of 5 μl min −1 for 6 min. Analytical separations were performed on a 75 μm × 250 mm column packed with 1.8 μm HSS T3 C18 particles (Waters Corporation). Mobile phase A was water with 0.1% formic acid, and mobile phase B was acetonitrile with 0.1% formic acid (Fisher). Water and acetonitrile were Optima LC-MS grade, and all other chemicals were ACS reagent grade or higher. At a flow rate of 400 nl min −1 , a 90 min gradient from 5 to 40% B was used to separate the peptides. The outlet of the column was connected to a silica electrospray emitter (New Objective, Inc) operated at +2.6 kV. The Synapt G2 mass spectrometer analyser operated at a resolution of ∼ 20,000 in ion-mobility data-independent acquisition (IMS-MS E ) mode. Parent ions were scanned from 50 to 2,000 m / z over 0.6 s at 4 eV. MS E scans to collect fragment ion data were performed by ramping collision energy from 27 to 50 eV over 0.6 s. Peptide data processing Peptide data were initially processed using ProteinLynx Global Server 2.5.2 (Waters Corporation) and deconvoluted tandem mass spectrometry spectra were searched against a database of known yeast proteins from Uni-Prot ( www.uniprot.org ) protein knowledgebase with a 1 × reversed sequence appended and 100% false discovery rate. These results were then imported into Scaffold 4.2.0 (Proteome Software, Portland, OR) with a 4.9% protein false discovery rate and a minimum of three peptides for protein identification. Peptides matching multiple proteins were exclusively assigned to the protein with the most evidence. The spectral counts for each peptide assigned to a protein were summed to give the quantitative value of the protein. The value was normalized by multiplying the average total number of spectra, for each biological sample, divided by the total number of spectra for each analytical replicate. Bovine serum albumin was used as the standard to covert the average intensity of the top 3 ‘best-flier’ peptides for each proteins to moles using the method of Silva [41] . The quantified amounts (fmol) for proteins identified in two of the three biological replicates were averaged and a Fisher’s exact test was performed between WT cells and cells that display error-prone transcription. Proteins that contained a P value<0.050 between the two samples and a fold change >1.5 were considered differentially expressed. Spotting assay Single colonies were picked up from glucose plates and inoculated into medium containing 3% raffinose. Cells were grown overnight, and diluted 10-fold in fresh medium containing 3% raffinose. After 4.5 h of growth, the cells were diluted to OD 0.2, and spotted on plates containing either galactose or glucose. Fluorescence microscopy Single colonies were inoculated in YAPD, grown overnight and then diluted in fresh YAPD the next morning. Cells were grown into log-phase, collected and imaged using a Nikon Lumencore microscope at × 250 magnification, or a Zeiss confocal microscope at × 160 magnification, in synthetic complete buffer using an light-emitting diode lamp for illumination and standard GFP and RFP filters for data collection. All images were collected with Metamorph and Zen software, and analysed in ImageJ. Growth assays Single colonies were inoculated in YAPD, grown overnight and then diluted in fresh YAPD the next morning. Cells were grown into log-phase, collected and diluted to OD 0.001. These cells were then aliquoted into a 96-well plate, and grown for 24 h at 30 °C in a 96-well bioananalyser that recorded the OD in each well every 10 min. The growth rate of each genotype was monitored in triplicate or quadruplicate, starting from a unique, single colony. Drug treatments Cells were grown in YAPD, YAPD containing 0–800 μM MG-132, or YAPD containing 0–800 μM and 200 μM PMSF. To determine the effect of these drugs on the cells, we grew the cells for 9 h and then compared the OD of cells grown in YAPD with the OD of cells grown in YAPD plus drugs. Transcription fidelity measurements Transcription fidelity assays were performed as previously reported [9] . Briefly, transcriptional errors on a tract of 10 cytosines result in accurate synthesis of the Cre-recombinase gene, which excises a drug-resistance gene inserted into an artificial intron in the ADE6 gene, ade6-AI2floxkanMX. The kanMX gene is flanked by two lox sites. Cre-recombinase excises the kanMX gene generating the functional ADE6-AI2lox allele. In yeast that carry an ade2 mutation, the Cre-mediated switch from ade6-AI2flox::kanMX to ADE6-AI2lox results in a colony colour change from white to red. During replicative lifespan experiments, virgin cells containing the reporter construct were selected and the transcriptional error rate of each cell was determined as a function of their age. For example, if a cell gave birth to a total of 20 daughters, and a transcription error occurred at daughter 17, then the error occurred at 85% of its lifespan (diploid cross between GRY3337 and GRY3724). During chronological lifespan assays, cells were grown into stationary phase for 48 h in YAPD (day 0) and aged for extended periods of time, while the number of CFUs was determined every 3 days (diploid cross between GRY3337 and GRY3724). We then recorded the number of colonies that emerged to monitor the lifespan and recorded the colonies that were either half red or a quarter red. These patterns result from a single, aged mother cell that committed a transcription error either during the first (half red) or second cell division (quarter red) after plating. These numbers were then used to calculate the error rate per 100 cell divisions. How to cite this article: Vermulst, M. et al. Transcription errors induce proteotoxic stress and shorten cellular lifespan. Nat. Commun. 6:8065 doi: 10.1038/ncomms9065 (2015).